Room-temperature chemical synthesis of C2 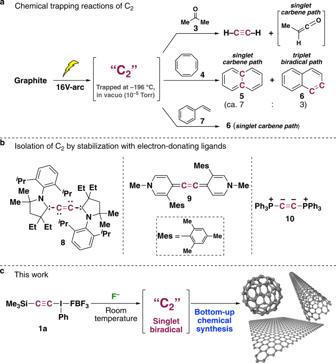Fig. 1: Previous experimental work on C2and our synthesis of C2at low temperature in a flask. aChemical trapping of C2generated by a carbon arc.bIsolation of C2stabilized by potent electron-donating ligands.cOur chemical synthesis of C2at ambient temperature under normal pressure by utilizing hypervalent alkynyl-λ3-iodane1a. Diatomic carbon (C 2 ) is historically an elusive chemical species. It has long been believed that the generation of C 2 requires extremely high physical energy, such as an electric carbon arc or multiple photon excitation, and so it has been the general consensus that the inherent nature of C 2 in the ground state is experimentally inaccessible. Here, we present the chemical synthesis of C 2 from a hypervalent alkynyl-λ 3 -iodane in a flask at room temperature or below, providing experimental evidence to support theoretical predictions that C 2 has a singlet biradical character with a quadruple bond, thus settling a long-standing controversy between experimental and theoretical chemists, and that C 2 serves as a molecular element in the bottom-up chemical synthesis of nanocarbons such as graphite, carbon nanotubes, and C 60 . Diatomic carbon (C 2 ) exists in carbon vapor, comets, the stellar atmosphere, and interstellar matter, but although it was discovered in 1857 [1] , it has proven frustratingly difficult to characterize, since C 2 gas occurs only at extremely high temperatures (above 3500 °C) [2] . 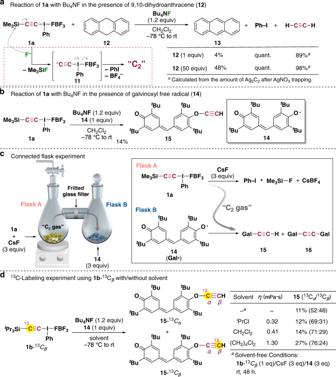Fig. 2: Chemical trapping of C2synthesized at low temperature. aReaction of1awith Bu4NF in the presence of 9,10-dihydroanthracene (12).bReaction of1awith Bu4NF in the presence of galvinoxyl free radical14.cConnected-flask experiment.d13C-Labeling experiments using1b-13Cβ. Considerable efforts have been made to generate/capture C 2 experimentally and to measure its physicochemical properties. The first successful example of artificial generation of C 2 , which was confirmed spectroscopically, involved the use of an electric carbon arc under high vacuum conditions [3] . Subsequent chemical trapping studies pioneered by Skell indicated that C 2 behaves as a mixture of singlet dicarbene and triplet biradical states in a ratio of 7:3 to 8:2 (Fig. 1a ) [4] , [5] , [6] , [7] . Multiple photon dissociation of two-carbon small molecules (acetylene, ethylene, tetrabromoethylene, etc.) by infrared or UV irradiation in the gas phase was also developed to generate C 2 , but this photo-generated C 2 also exhibited several electronic states [8] . Recently, other approaches for the isolation of C 2 have been reported, using potent electron-donating ligands to stabilize C 2 by means of dative interactions (L:→C 2 ←:L), but such stabilized complexes no longer retain the original character of C 2 (Fig. 1b ) [9] , [10] , [11] , [12] . Instead, theoretical/computational simulation has been applied recently, and the results indicated that C 2 has a quadruple bond with a singlet biradical character in the ground state [13] , [14] . Fig. 1: Previous experimental work on C 2 and our synthesis of C 2 at low temperature in a flask. a Chemical trapping of C 2 generated by a carbon arc. b Isolation of C 2 stabilized by potent electron-donating ligands. c Our chemical synthesis of C 2 at ambient temperature under normal pressure by utilizing hypervalent alkynyl-λ 3 -iodane 1a . Full size image These various theoretical and experimental findings have sparked extensive debate on the molecular bond order and electronic state of C 2 in the scientific literature, probably because of the lack of a method for the synthesis of ground-state C 2 . Here, we present a straightforward room-temperature/pressure synthesis of C 2 in a flask. We show that C 2 generated under these conditions behaves exclusively as a singlet biradical with quadruple bonding, as predicted by theory. We also show that spontaneous, solvent-free reaction of in situ generated C 2 under an argon atmosphere results in the formation of graphite, carbon nanotubes (CNTs), and fullerene (C 60 ) at room temperature. This not only represents a bottom-up chemical synthesis of nanocarbons at ordinary temperature and pressure, but it also provides experimental evidence that C 2 may serve as a key intermediate in the formation of various carbon allotropes (Fig. 1c ). Chemical synthesis of C 2 The key strategy underlying the present achievement is the use of hypervalent iodane chemistry [15] , [16] , [17] , aiming to utilize the phenyl-λ 3 -iodanyl moiety as a hyper-leaving group (ca. 10 6 times greater leaving ability than triflate (–OSO 2 CF 3 ), a so-called super-leaving group) [18] . We designed [ β -(trimethylsilyl)ethynyl](phenyl)-λ 3 -iodane 1a [19] , in the expectation that it would generate C 2 upon desilylation of 1a with fluoride ion to form anionic ethynyl-λ 3 -iodane 11 , followed by facile reductive elimination of iodobenzene. Gratifyingly, exposure of 1a to 1.2 equivalents of tetra- n -butylammonium fluoride (Bu 4 NF) in dichloromethane resulted in smooth decomposition at −30 °C with the formation of acetylene and iodobenzene, indicating the generation of C 2 ! However, all attempts to capture C 2 with a range of ketones and olefins, such as acetone ( 3 ), 1,3,5,7-cyclooctatetraene ( 4 ), styrene ( 7 ), and 1,3,5-cycloheptatriene, failed, though they smoothly reacted with arc-generated C 2 on an argon matrix at −196 °C [3] , [4] , [5] , [20] . These findings immediately suggested that the putative C 2 synthesized here at −30 °C has a significantly different character from C 2 generated under high-energy conditions (Supplementary Fig. 1 ). Experimental evidence for singlet biradical character Taking account of the fact that quantum chemical calculations suggest a relatively stable singlet biradical C 2 with quadruple bonding in the ground state, we next examined an excellent hydrogen donor. 9,10-Dihydroanthracene has very weak C–H bonds (bond dissociation energy of 12 : 76.3 kcal mol −1 vs CH 2 Cl 2 : 97.3 kcal mol −1 ) [21] , [22] that might effectively trap the putative singlet biradical C 2 . When 12 was added to the reaction mixture, anthracene ( 13 ) was obtained accompanied with the formation of acetylene (Fig. 2a ), which clearly suggests that the generation of C 2 and subsequent hydrogen abstraction from 12 gave acetylene. The formation of acetylene was confirmed by Raman spectroscopy after AgNO 3 trapping, and the amount of acetylene was estimated by the quantitative analysis of Ag 2 C 2 thus generated (Supplementary Fig. 2 ). These results strongly support the relatively stable (singlet) biradical nature of our C 2 , in accordance with the theoretical calculations. Thus, we turned our attention to the galvinoxyl free (stable) radical 14 in order to trap C 2 directly. To our delight, O -ethynyl ether 15 was obtained in 14% yield, accompanied with the formation of acetylene (84%) (Fig. 2b ). The structure of 15 was fully characterized by 1 H/ 13 C NMR spectra: an upfield-shifted acetylenic proton was seen at 1.78 ppm in the 1 H NMR, as well as considerably separated 13 C NMR chemical shifts of two acetylenic carbons (C α : 90.4 ppm and C β : 30.0 ppm), clearly indicating the presence of an ethynyl ether unit (e.g., ethynyl ethyl ether, C α : δ 88.2 ppm; C β : δ 22.0 ppm) [23] . In solution, di-galvinoxyl alkyne 16 was undetectable or barely detectable even when excess amounts of 14 were used, though 15 was obtained as almost the sole product in all cases. On the other hand, when we performed the trapping reaction in the presence of two equivalents of 14 under solvent-free conditions, 16 was clearly observed by atmospheric pressure chemical ionization (APCI) mass spectrometry (MS), although in very small quantity (Supplementary Fig. 3 ) [24] . These findings are consistent with the valence bond model of a singlet biradical species, according to which the energy barrier of the second hydrogen abstraction is lower by approximately 10 kcal/mol compared with the first hydrogen abstraction, which has to overcome the bonding energy of the singlet biradical [25] , [26] . It should be noted that the O -phenylated product was not formed at all, excluding alternative single electron transfer pathways, such as those via ethynyl(phenyl)-λ 2 -iodanyl radical (Supplementary Fig. 4 ) [27] . Fig. 2: Chemical trapping of C 2 synthesized at low temperature. a Reaction of 1a with Bu 4 NF in the presence of 9,10-dihydroanthracene ( 12 ). b Reaction of 1a with Bu 4 NF in the presence of galvinoxyl free radical 14 . c Connected-flask experiment. d 13 C-Labeling experiments using 1b - 13 C β . Full size image In order to obtain more direct information about the generation of C 2 “gas,” we designed a connected-flask, solvent-free experiment (Fig. 2c ): a solvent-free chemical synthesis of C 2 using 1a with three equivalents of CsF was carried out in one of a pair of connected flasks (Flask A), and three equivalents of 14 was placed in the other flask (Flask B). The reaction mixture in Flask A was vigorously stirred at room temperature for 72 h under argon. As the reaction proceeds in Flask A, generated C 2 gas should pass from Flask A to Flask B. Indeed, the color of 14 in Flask B gradually changed from deep purple to deep brown as the reaction progressed. After 72 h, the formation of 15 and 16 was confirmed by APCI–MS analysis of the residue in Flask B. We then performed a 13 C-labeling experiment using 1b - 13 C β , which was synthesized from H 3 13 C –I in eight steps [28] , [29] . Treatment of 1b - 13 C β (99% 13 C) with Bu 4 NF in the presence of 14 in CH 2 Cl 2 gave a mixture of 15 - 13 C α and 15 - 13 C β , suggesting that C 2 is generated before the O -ethynyl bond-forming reaction with 14 (Fig. 2d ). The observed O – 13 C/ 12 C selectivity (71:29) may be related to very fast radical pairing between C 2 and 14 prior to ejection of iodobenzene from the solvent cage [30] . We also carried out 13 C-labeling experiments using 1b - 13 C β in solvents of different viscosities (η). The observed O – 13 C/ 12 C selectivity decreased as the viscosity decreased, and the regioselectivity was almost lost (52:48) under solvent-free conditions. Similarly, the O – 13 C/ 12 C selectivity was 51:49 in the connected-flask experiment. All these findings rule out stepwise addition/elimination mechanisms (Supplementary Fig. 5 ). Role as molecular element of nanocarbons Given that C 2 generated at room temperature or below behaves exclusively as a singlet biradical, as theoretically predicted for the ground state, we examined whether this ground-state C 2 would serve as a molecular element for the formation of various carbon allotropes. Today, nanocarbons such as graphene, CNTs, and fullerenes, in which sp 2 carbon takes the form of a planar sheet, tube, ellipsoid, or hollow sphere, are at the heart of nanotechnology [31] . But, in contrast with the rapid growth of their practical applications, the mechanisms of their formation remain unclear. Various models and theories for the growth of carbon allotropes have been proposed, most of which include the addition/insertion of C 2 into a growing carbon cluster as a key step [32] , [33] , [34] , [35] , [36] , [37] , [38] , [39] . However, this idea lacks experimental verification. To investigate this issue, we examined the solvent-free reaction of the present singlet biradical C 2 in order to avoid hydrogen quenching. Notably, simple grinding of CsF and 1.5 equivalents of 1a in a mortar and pestle at ambient temperature for 10 min under an argon atmosphere resulted in the formation of a dark-brown solid containing various carbon allotropes, as determined by resonance Raman spectroscopy (Supplementary Fig. 6 ), matrix-assisted laser desorption ionization time-of-flight (MALDI-TOF) MS (Fig. 3a ) and electrospray ionization (ESI) MS (Supplementary Fig. 8 ). Careful examination of the Raman spectra and high-resolution transmission electron micrograph (HRTEM) images indicated that high-quality graphite with few defects and an interlayer distance of 0.33 nm (Fig. 4a–c ) and amorphous carbon (ca. 80–30% yields) had been mostly synthesized (Supplementary Fig. 6a ), together with very small amounts of C 60 (Fig. 3a and Supplementary Figs. 8 , 9a , and 10 – 12 ) and CNTs/carboncones (Fig. 4d and Supplementary Figs. 6b , and 7 ) [40] , [41] . The chemical synthesis of double/triple-walled CNTs/carboncones has never previously been reported. We did not observe any peaks attributable to larger fullerenes, such as C 70 , C 76 , C 78 , and C 84 . This specificity may reflect the ambient temperature/pressure condition, as the electric carbon arc method generally affords a fearsome mixture of carbon allotropes. Fig. 3: Solvent-free reaction of in situ generated C 2 in a mortar at room temperature leads to spontaneous formation of carbon allotropes. MALDI-TOF mass spectra of a Ground 1a and CsF. b Ground 1a and CsF in the presence of CuCl (1.0 equiv). c Ground 1b - 13 C β and CsF. Full size image Fig. 4: Raman spectra and HRTEM images (and their power spectra) of carbon allotropes. a Raman spectrum of graphite-containing sample. b HRTEM image and power spectrum of graphite-containing sample corresponding to the (002) lattice plane. c HRTEM image and power spectrum of graphite-containing sample corresponding to the (100) lattice plane. d HRTEM image of carbon nanotube-containing sample. Full size image By using 1b - 13 C β , we further confirmed that C 60 is synthesized from C 2 . Grinding of 1b - 13 C β with CsF under the same reaction conditions as above afforded C 60 - 13 C 30 , which was detected by means of MALDI-TOF and ESI MS, while nonlabeled C 60 was not detected at all (Fig. 4c and Supplementary Fig. 9b ). The formation of this unique fullerene is solid evidence for the role of C 2 , as its occurrence probability in nature is extremely small [(0.01) 30 ]. When CuCl was added to the reaction mixture (which can stabilize alkynyl radical termini), a mixture of various fragments of polyynes –[C≡C] n – with different chain lengths was observed by MALDI-TOF MS (Fig. 4b ). Such peaks were not observed from authentic C 60 , graphite, and SWCNTs (<ca. 7 nm in diameter) under the same measurement conditions. Lagow et al. proposed that linear acetylenic carbon biradicals (•[C≡C] n •) are a key intermediate/precursor for the formation of C 60 , and our results seem to support this view [34] , [39] . In conclusion, we have generated C 2 at ordinary temperature and pressure. Further, we have established that it has a singlet biradical character at low temperature, settling a long-standing difference of opinion between experimental and theoretical chemists. We also observed spontaneous formation of carbon allotropes such as graphite, CNTs, carboncones, amorphous carbon, and C 60 from C 2 at ambient temperature, providing the first experimental support for the generally held belief that the formation mechanism of nanocarbons involves the addition/insertion of C 2 into a growing carbon cluster as a key step. This is also represents the first chemical synthesis of nanocarbons at ordinary temperature and pressure from C 2 in the ground state. Easy synthetic access to in situ generated C 2 should be helpful in opening up additional areas of chemistry and materials science, including further studies on the hot topic of the growth mechanisms of bottom-up synthesis of nanocarbons from C 2 . General procedure for solid-state reaction of alkynyl-λ 3 -iodane 1a with CsF Alkynyl-λ 3 -iodane 1a (71 mg, 0.15 mmol) and cesium fluoride (15 mg, 0.10 mmol) were gently mixed in an agate mortar under argon, and the mixture was ground for 10 min. The color of the reaction mixture gradually changed from yellowish white to dark brown during the grinding process. The solid residue was treated with excess t- BuOK in order to remove remaining 1a , and then carefully extracted with toluene (ca. 1 mL × 3) and the combined organic phase was analyzed by MALDI-TOF (Fig. 4a and Supplementary Fig. 12 ) and ESI MS (Supplementary Figs. 8 and 9a ). LC-UV analysis was performed with TSKgel ODS-120T (250 × 4.6 mm) using toluene/MeCN = 50/50 as an eluent (Supplementary Fig. 11 ). LC-MS analysis was performed with Shim-Pack GIST-HP C18 (150 × 2.1 mm) using toluene/MeCN = 60/40 as an eluent (Supplementary Fig. 9 ). Yield of fullerene C 60 was determined to be 4.0 × 10 −5 % by using an external standard method. As shown below, a linear calibration curve was obtained for toluene solutions of C 60 over the concentration range from 1 to 60 ppb (1, 3, 6, 10, 30, and 60 ppb); the correlation coefficient was R 2 = 0.99 (Supplementary Fig. 18 ). In a separate experiment, after toluene extraction, the reaction mixture was washed several times with water, dispersed in a small amount of ethanol, and dried on a stainless steel plate, which was analyzed by Raman spectroscopy (Supplementary Fig. 6a ). Further oxidative treatment in order to remove amorphous carbon from the reaction mixture was carried out as described below. Oxidative treatment with hydrogen peroxide To the reaction mixture (8.0 mg) obtained above experiment was added an excess of 20% H 2 O 2 aqueous solution (ca. 8 mL), and the mixture was heated at 100 °C for 24 h [42] . After cooling, the mixture was centrifuged (4000 rpm, 10 min) and the supernatant was removed. The residue was washed several times with deionized water and then analyzed by Raman spectroscopy (Fig. 4a and Supplementary Fig. 6b ) and HRTEM (Fig. 4b, c ). Oxidative treatment with nitric acid To the reaction mixture (48 mg) obtained above experiment was added an excess of 3.2 M HNO 3 aqueous solution (ca. 48 mL) and the mixture was heated at 100 °C for 24 h [43] . After cooling, the mixture was filtered and washed with deionized water, followed by four times with 4 M NaOH aqueous solution and finally with deionized water. The residue was then analyzed by Raman spectroscopy and HRTEM (Fig. 4d and Supplementary Fig. 7 ). Experimental data For experimental procedures and spectroscopic data of the compounds, see Supplementary Information . 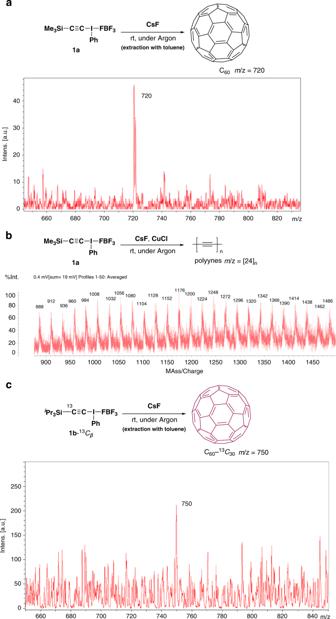Fig. 3: Solvent-free reaction of in situ generated C2in a mortar at room temperature leads to spontaneous formation of carbon allotropes. MALDI-TOF mass spectra ofaGround1aand CsF.bGround1aand CsF in the presence of CuCl (1.0 equiv).cGround1b-13Cβand CsF. 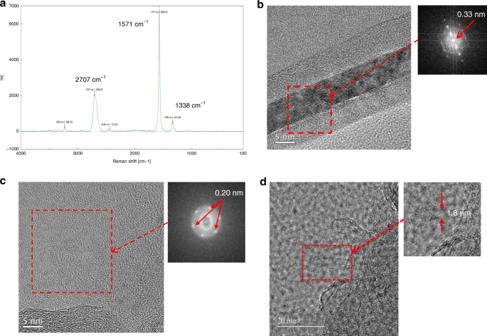Fig. 4: Raman spectra and HRTEM images (and their power spectra) of carbon allotropes. aRaman spectrum of graphite-containing sample.bHRTEM image and power spectrum of graphite-containing sample corresponding to the (002) lattice plane.cHRTEM image and power spectrum of graphite-containing sample corresponding to the (100) lattice plane.dHRTEM image of carbon nanotube-containing sample. For general procedures for alkynyl-λ 3 -iodanes 1b - 13 C β and trapping reactions, see Supplementary Methods and Supplementary Figs. 1 and 2 . For Raman, HRTEM, ESI mass, LC-ESI mass, UV–Vis, LC-UV chromatograms, and MALDI-TOF mass spectra of a sample obtained by a solvent-free reaction, see Supplementary Figs. 6 – 12 . For NMR spectra see Supplementary Figs. 13 – 17 .